AnArabidopsisPWI and RRM motif-containing protein is critical for pre-mRNA splicing and ABA responses The phytohormone abscisic acid (ABA) is important for growth, development and stress responses in plants. Recent research has identified ABA receptors and signalling components that regulate seed germination and stomatal closure. However, proteins that regulate ABA signalling remain poorly understood. Here we use a forward-genetic screen to identify rbm25-1 and rbm25-2 , two Arabidopsis mutants with increased sensitivity to growth inhibition by ABA. Using RNA-seq, we found that RBM25 controls the splicing of many pre-mRNAs. The protein phosphatase 2C HAB1, a critical component in ABA signalling, shows a dramatic defect in pre-mRNA splicing in rbm25 mutants. Ectopic expression of a HAB1 complementary DNA derived from wild-type mRNAs partially suppresses the rbm25-2 mutant phenotype. We suggest that RNA splicing is of particular importance for plant response to ABA and that the splicing factor RBM25 has a critical role in this response. The phytohormone abscisic acid (ABA) is critical for many processes in the life cycle of plants, such as the promotion of seed maturation, establishment and maintenance of seed dormancy, regulation of stomatal aperture and adaptation to environmental stresses [1] , [2] , [3] . On exposure to environmental stresses, plants rapidly increase their ABA content as a result of increased ABA synthesis, decreased ABA catabolism, decreased formation of inactive ABA conjugates, or a combination of these factors [4] . The de novo biosynthesis of ABA is through the cleavage of a C 40 carotenoid precursor, followed by the conversion of the intermediate xanthoxin to ABA via ABA aldehyde [2] . The cleavage step catalysed by a 9- cis epoxycarotenoid dioxygenase (NCED) has generally been considered the rate-limiting step in the pathway [4] , [5] . Wang et al . [6] found that CED1 (for NCED defective 1), which is a putative α/β hydrolase domain-containing protein and is allelic to the BODYGUARD gene that is essential for cuticle biogenesis, plays an important role in regulating the expression of NCED3 and genes encoding other signalling components downstream of ABA biosynthesis. Following ABA biosynthesis, multiple signal transduction pathways, which amplify the primary signal produced when ABA binds to its receptors, are required to control the ABA-regulated adaptive responses. These adaptive responses include stomatal closure (which allows the plant to conserve water), the accumulation of compatible osmolytes such as proline [7] , and the differential expression of a wide array of stress-responsive genes [8] , [9] . The core ABA signal transduction pathway is mediated by receptors in the PYR/PYL/RCAR family, which, on binding to ABA, inhibit the type 2C protein phosphatases (PP2Cs) such as ABI1, ABI2 and HAB1 (refs 3 , 10 , 11 , 12 ). The PP2Cs are negative regulators of the ABA signalling pathway [13] , [14] . Inhibition of the PP2Cs leads to the activation of protein kinases in the sucrose non-fermenting related kinase 2 (SnRK2) family. In the absence of ABA, the PP2Cs can directly inactivate SnRK2 kinases by dephosphorylating a critical amino acid residue in their kinase activation loop [15] , [16] . These kinases are required for the subsequent regulation of the activities of downstream effectors in ABA signalling. Since the three SnRK2 kinases, SnRK2.2, SnRK2.3 and SnRK2.6, control virtually all of the ABA responses in plants, the substrate proteins of the SnRK2s function as the downstream effectors of ABA responses [17] . The best known of the substrates include several transcription factors and ion channels [18] , [19] , [20] , [21] . The basic leucine zipper family transcription factors such as ABI5 and other ABA response factors or ABA-responsive element-binding factors (AREBs) control the transcription of ABA-responsive genes [18] , [20] . The ion channels such as the slow anion channel SLAC1 and the potassium channel KAT1 are critical for guard cell regulation by ABA [19] , [21] , [22] , [23] , [24] . Recent phosphoproteomics studies identified dozens of additional substrate proteins of the SnRK2s including several proteins with potential roles in RNA processing and proteins involved in chloroplast function [25] , [26] . These newly identified substrate proteins are potential effectors of ABA signalling, although their functions in ABA responses are largely unknown. To identify cellular factors important for ABA responses, particularly ABA responses in leaf development, we conducted a genetic screen in Arabidopsis thaliana for mutants with defective leaf greening response to ABA treatment. We report here that roa1 ( regulator of ABA response ) mutants are hypersensitive to ABA (HAB) as indicated by impaired leaf greening in response to ABA. The ROA1/RBM25 locus defines a splicing factor required for the splicing of transcripts of many genes including those involved in ABA signal transduction pathways. Our work has revealed a critical role of pre-mRNA splicing in ABA responses in plants. roa1 mutants are hypersensitive to ABA Identification of a large number of mutants defective in seed germination or guard cell movements has led to the discovery of genes involved in ABA biosynthesis and its downstream signalling events [3] . High levels of ABA inhibit plant growth and development and cause leaves to become pale or yellow [27] , [28] . The cellular factors controlling these processes are poorly understood. To identify critical regulators for ABA responses at the seedling growth stage, we screened an A. thaliana transfer DNA (T-DNA) insertion population with known integration sites (the SALK collection from ABRC) for mutants with increased sensitivity to exogenous ABA in the growth medium in terms of root growth and leaf yellowing. A similar screen was performed with an in-house generated T-DNA insertional population in a TOUCH 4 promoter:luciferase reporter line [29] ( pTCH4:LUC ). These mutants were designated as roa . The roa1-1 (SALK_064472 from the SALK collection) and roa1-2 (from the pTCH4:LUC population) mutants were chosen for in-depth characterization ( Supplementary Fig. 1a ). To compare roa1-1 and roa1-2 side-by-side, roa1-2 was backcrossed with Col-0 and roa1-2 allele without the pTCH4:LUC transgene was obtained. In the absence of exogenous ABA, roa1-1 and roa1-2 seedlings do not exhibit obvious growth defects ( Fig. 1a ). However, after being transferred to media supplemented with 5 μM ABA, the newly emerged leaves in roa1-1 and roa1-2 seedlings are yellow, whereas all of the leaves in the wild-type seedlings are green ( Fig. 1a ). The mutants also had reduced primary root elongation in response to 5 μM ABA ( Fig. 1a,b ).There is substantially less accumulation of chlorophylls in ABA-treated roa1-1 and roa1-2 leaves ( Fig. 1a,c ). Genetic analysis showed that both roa1-1 and roa1-2 mutations are recessive and are caused by mutations in a single nuclear gene ( Supplementary Data 1 ). Pair-wise crosses between roa1-1 and roa1-2 suggested that the roa1-1 and roa1-2 mutations are allelic to each other ( Fig. 1d ). 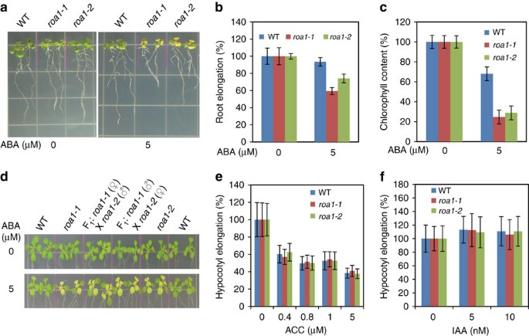Figure 1: Sensitivity ofroa1mutants to ABA, ethylene precursor ACC and auxin. Five-day-old seedlings grown in MS medium were transferred to MS medium containing 0 or 5 μM ABA and grown for an additional 14-day period (fora–d). (a)roa1mutants are hypersensitive to ABA. (b) Root elongation of seedlings shown ina. Root elongation was measured and is shown as a percentage relative to growth on normal MS medium. (c) Chlorophyll content of seedlings shown ina. (d) Sensitivity of F1seedlings from pair-wised crosses betweenroa1-1androa1-2to ABA. Hypocotyl elongation of wild-type,roa1-1androa1-2seedlings (fore–f). Seeds were germinated directly on medium containing various levels of ACC (ine; in darkness) or indole-3-acetic acid (inf; 8-h light (80 μmol m−2s−1) and 16-h dark cycle). Seedlings were allowed to grow for an additional 3-day (ine) or 5-day period (inf) after germination. Values represent mean±s.d. (n=20 inb, 8–10 pools of 4–5 seedlings inc, 49–135 ineand 89–125 inf). Figure 1: Sensitivity of roa1 mutants to ABA, ethylene precursor ACC and auxin. Five-day-old seedlings grown in MS medium were transferred to MS medium containing 0 or 5 μM ABA and grown for an additional 14-day period (for a – d ). ( a ) roa1 mutants are hypersensitive to ABA. ( b ) Root elongation of seedlings shown in a . Root elongation was measured and is shown as a percentage relative to growth on normal MS medium. ( c ) Chlorophyll content of seedlings shown in a . ( d ) Sensitivity of F 1 seedlings from pair-wised crosses between roa1-1 and roa1-2 to ABA. Hypocotyl elongation of wild-type, roa1-1 and roa1-2 seedlings (for e – f ). Seeds were germinated directly on medium containing various levels of ACC (in e ; in darkness) or indole-3-acetic acid (in f ; 8-h light (80 μmol m −2 s −1 ) and 16-h dark cycle). Seedlings were allowed to grow for an additional 3-day (in e ) or 5-day period (in f ) after germination. Values represent mean±s.d. ( n =20 in b , 8–10 pools of 4–5 seedlings in c , 49–135 in e and 89–125 in f ). Full size image To investigate whether the roa1-1 and roa1-2 mutations alter plant responses to other plant hormones or abiotic stress, we examined the responses of roa1-1 and roa1-2 plants to heat stress and two additional hormones. Sensitivity of the soil-grown roa1-1 and roa1-2 plants at both vegetative and reproductive stages to heat stress is not altered when they are compared with the wild-type plants ( Supplementary Fig. 1b ). We used the precursor of ethylene biosynthesis, 1-amino-cyclopropane-1-carboxylic acid (ACC), to examine the effect of ethylene on hypocotyl elongation of dark grown roa1-1 and roa1-2 seedlings. Hypocotyl elongation of roa1-1, roa1-2 and wild-type seedlings was equally inhibited by exogenous application of ACC ( Fig. 1e ; Supplementary Fig. 1c ). We further examined effects of auxin on hypocotyl and root elongation of roa1-1 and roa1-2 seedlings. roa1-1 and roa1-2 seedlings essentially responded to the same extent to indole-3-acetic acid in the growth media ( Fig. 1f ; Supplementary Fig. 1d,e ). Therefore, while ROA1 may be involved in the response to stresses and hormones other than ABA, we find no evidence of its involvement in the response to auxin, ethylene or heat. ROA1 encodes a PWI and RRM motif-containing protein Although roa1-1 /SALK_064472 was annotated as having a T-DNA insertion in the At1g60200 gene, we could not find any T-DNA insertion in this gene. We carried out thermal asymmetric interlaced PCR (TAIL-PCR) analysis and identified a T-DNA insertion downstream of At1g60200 in roa1-1 ( Fig. 2a ). Although roa1-2 also came from a T-DNA mutant population, there is no T-DNA insertion in roa1-2 . To identify the gene responsible for the roa1-1 and roa1-2 mutant phenotypes, we prepared mapping populations by crossing roa1-1 and roa1-2 mutants with Landsberg erecta wild-type plants and performed map-based cloning for the ROA1 locus. Genetic mapping pinpointed ROA1 to a genomic region that contains the At1g60200 gene. In the roa1-1 mutant, we identified a single nucleotide substitution in At1g60200 , and this substitution changes alanine at position 899 to valine in the deduced polypeptide ( Fig. 2a,b ). The roa1-2 mutation also has a single nucleotide substitution in At1g60200 , which results in the change of glutamine at position 570 to a premature stop codon in the deduced polypeptide ( Fig. 2a,b ). We confirmed the ROA1 gene is At1g60200 by functional complementation analysis. The wild-type At1g60200 gene driven by its native promoter complemented the roa1-1 and roa1-2 mutant phenotype ( Fig. 2d,e ). ROA1 expression is severely disrupted in roa1-1 , possibly due to the T-DNA insertion downstream of ROA1 ( Fig. 2f ). 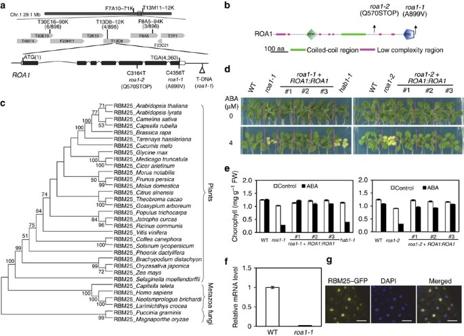Figure 2: Molecular cloning ofROA1. (a) Map-based cloning ofROA1. Structure of theROA1gene and positions of theroa1-1androa1-2mutations are indicated. Filled boxes and empty boxes indicate exons and untranslated regions, respectively; the solid lines between boxes indicate introns. Positions are relative to translation start sites. (b) Structure of ROA1. Motifs are predicted by the SMART database. (c) Phylogenetic tree of RBM25 and its close orthologues from other organisms. The protein identities are the same as defined inSupplementary Fig. 2. The Bootstrap consensus tree was generated with MEGA6 (ref.69). Protein sequences of RBM25 and its orthologues were aligned by MUSCLE and the Bootstrap consensus phylogenetic tree was reconstructed by the statistical method maximum likelihood using the Jones–Taylor–Thornton (JTT) model with a Bootstrap of 1000. Cut-off value for consensus tree is 50%. (d) Gene complementation analysis. (e) Chlorophyll content in plants shown ind. (f) Relative transcript levels ofROA1in WT androa1-1plants as determined by qRT–PCR analysis. (g) Nuclear localization of the RBM25–GFP fusion protein. Scale bars, 2.5 μm. Values represent mean±s.d. (n=8 ine; 4 inf). Figure 2: Molecular cloning of ROA1 . ( a ) Map-based cloning of ROA1 . Structure of the ROA1 gene and positions of the roa1-1 and roa1-2 mutations are indicated. Filled boxes and empty boxes indicate exons and untranslated regions, respectively; the solid lines between boxes indicate introns. Positions are relative to translation start sites. ( b ) Structure of ROA1. Motifs are predicted by the SMART database. ( c ) Phylogenetic tree of RBM25 and its close orthologues from other organisms. The protein identities are the same as defined in Supplementary Fig. 2 . The Bootstrap consensus tree was generated with MEGA6 (ref. 69 ). Protein sequences of RBM25 and its orthologues were aligned by MUSCLE and the Bootstrap consensus phylogenetic tree was reconstructed by the statistical method maximum likelihood using the Jones–Taylor–Thornton (JTT) model with a Bootstrap of 1000. Cut-off value for consensus tree is 50%. ( d ) Gene complementation analysis. ( e ) Chlorophyll content in plants shown in d . ( f ) Relative transcript levels of ROA1 in WT and roa1-1 plants as determined by qRT–PCR analysis. ( g ) Nuclear localization of the RBM25–GFP fusion protein. Scale bars, 2.5 μm. Values represent mean±s.d. ( n =8 in e ; 4 in f ). Full size image ROA1 encodes a putative PWI and RRM motif-containing protein with similarities to the human RNA-binding protein 25 (HsRBM25) ( Fig. 2b,c ). Hereafter, we refer to ROA1 as Arabidopsis RBM25 and refer to roa1-1 and roa1-2 mutant alleles as rbm25-1 and rbm25-2 , respectively. Arabidopsis RBM25 shares substantial sequence similarity (50% over the RRM motif and 71% over the PWI motif) with the HsRBM25, which is known as a splicing factor [30] . Database searches revealed that RBM25 orthologues are present in other plant species including monocots (such as rice and maize) and dicots (such as soybean and tomato) ( Fig. 2c ; Supplementary Fig. 2 ). The last amino acid of RBM25 (changed to valine in rbm25-1 ) is conserved in nearly half of the plant RBM25 orthologues ( Supplementary Fig. 2 ). As expected of a putative splicing factor, the RBM25–green fluorescent protein (GFP) fusion protein driven by the RBM25 native promoter is localized in the nucleus of Arabidopsis root cells ( Fig. 2g ). RBM25 negatively controls ABA responses in early development Seed germination is sensitive to ABA and we were interested whether RBM25 plays a role in this process. rbm25-1 is slightly hypersensitive to exogenous ABA at the stage of seed germination ( Fig. 3a ) and is substantially hypersensitive to ABA in post-germination seedling development ( Fig. 3b,c ). This hypersensitivity to ABA was suppressed in three independent complementation lines of rbm25-1 ( Fig. 3a,b,c ), indicating that loss-of-function of RBM25 results in this phenotype. ABA is also known to induce stomatal closure on drought stress. We performed water loss assays with detached shoots of soil-grown rbm25 mutant plants to determine whether rbm25 mutations alter plant transpirational water loss. Transpirational water loss rates are the same between the wild-type and rbm25 mutants with or without exogenous application of ABA ( Fig. 3d ). These results suggest that rbm25 mutations do not alter stomatal responses to ABA. 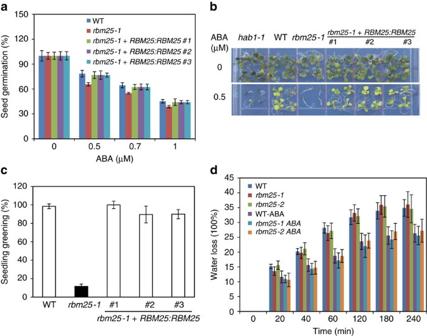Figure 3: Therbm25-1mutation alters sensitivity to ABA in seed germination and post-germination seedling development, but does not affect water loss rates. (a) Seed germination of WT,rbm25-1andrbm25-1complementation lines. Seeds (50–60 per genotype) were sown on surface of filter paper soaked with various levels of ABA. Seeds were considered germinated when radicles penetrate the seed coats. The percentage of seeds that had germinated 6 days after sowing was determined. (b) Post-germination seedling development of WT,rbm25-1andrbm25-1complementation lines subjected to 0 or 0.5 μM ABA. Photograph was taken 16 days after sowing seeds. (c) The percentage of green seedlings inb. Seedlings with fully developed green cotyledons and at least one true green leaf were considered green. (d) Shoots fromrbm25-1,rbm25-2and wild-type plants at the rosette stage were placed on weighing trays and allowed to dry slowly at constant temperature (25 °C) and humidity (∼50%). Weights of shoots were determined over a 4-h period. ABA, 100 μM ABA for 3 h. Values are mean±s.d. (n=8 ina, 4 (number of MS medium plates containing 0 or 0.5 μM ABA; each plate has 30–40 seedlings per genotype inb, 8 ind). Figure 3: The rbm25-1 mutation alters sensitivity to ABA in seed germination and post-germination seedling development, but does not affect water loss rates. ( a ) Seed germination of WT, rbm25-1 and rbm25-1 complementation lines. Seeds (50–60 per genotype) were sown on surface of filter paper soaked with various levels of ABA. Seeds were considered germinated when radicles penetrate the seed coats. The percentage of seeds that had germinated 6 days after sowing was determined. ( b ) Post-germination seedling development of WT, rbm25-1 and rbm25-1 complementation lines subjected to 0 or 0.5 μM ABA. Photograph was taken 16 days after sowing seeds. ( c ) The percentage of green seedlings in b . Seedlings with fully developed green cotyledons and at least one true green leaf were considered green. ( d ) Shoots from rbm25-1 , rbm25-2 and wild-type plants at the rosette stage were placed on weighing trays and allowed to dry slowly at constant temperature (25 °C) and humidity ( ∼ 50%). Weights of shoots were determined over a 4-h period. ABA, 100 μM ABA for 3 h. Values are mean±s.d. ( n =8 in a , 4 (number of MS medium plates containing 0 or 0.5 μM ABA; each plate has 30–40 seedlings per genotype in b , 8 in d ). Full size image The rbm25-1 mutation alters transcript accumulation profiles We performed RNA-seq experiments to determine whether the rbm25-1 mutation affects transcript accumulation profiles and whether altered transcript accumulation profiles may help explain the increased sensitivity of rbm25-1 mutant to ABA treatment. We used the Illumina HiSeq 2500 System to sequence mRNA-seq libraries prepared from wild-type and rbm25-1 seedlings with three biological replicates and obtained a minimum of 14.7 million of pair-end clean sequence reads ( Supplementary Data 2 ). Compared with those in the wild-type, 106 genes displayed higher transcript levels (by at least 2-fold and with P <0.05), while 97 genes showed lower transcript levels in rbm25-1 under control conditions ( Fig. 4a,b ; Supplementary Data 2 ). The RNA-seq analysis also revealed that 185 genes displayed at least a 2-fold increase in transcript levels (relative to the wild type and with P <0.05), while 267 genes showed at least a 2-fold decrease in transcripts levels under 100 μM ABA treatment for 6 h ( Fig. 4a,b ; Supplementary Data 2 ). Furthermore, we found that there are 37 genes whose transcript levels are increased in rbm25-1 plants under control and ABA treatment conditions ( Fig. 4a ; Supplementary Data 2 ). Similarly, there are 37 genes whose transcript levels are reduced in rbm25-1 plants under control and ABA treatment conditions ( Fig. 4a ; Supplementary Data 2 ). The differentially expressed genes in rbm25-1 encode proteins with diverse functions, and a substantial number of these proteins have predicted functions in stress responses ( Fig. 4c ; Supplementary Data 2 ). For example, under ABA treatment, 62 genes with annotated functions associated with response to abiotic or biotic stimulus or response to stress showed increased transcript levels in rbm25-1 mutant seedlings ( Supplementary Data 2 ). This observation of large and preferential change in the expression of stress-related genes is consistent with the obviously more ‘stressed’ appearance of the mutant plants under ABA treatment ( Figs 1a and 3b ) as a result of their impaired ability to cope with ABA treatment. With quantitative reverse transcription–PCR (qRT–PCR) analysis, we confirmed that the expression of At5g65080 and At1g53490 is substantially reduced in rbm25 mutants, while expression of At4g33720 is increased in rbm25 mutants ( Fig. 4d ). At5g65080 encodes a MADS-box transcription factor. At1g53490 encodes a RING/U-box superfamily protein. At4g33720 encodes a CAP (cysteine-rich secretory proteins, Antigen 5 and Pathogenesis-related 1 protein) superfamily protein. 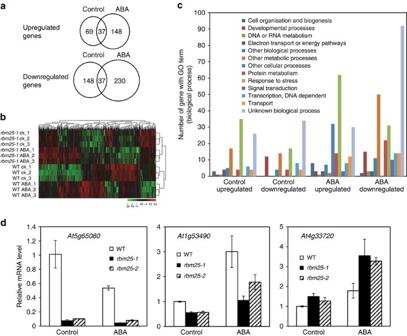Figure 4: Therbm25-1mutation causes disrupted gene expression as determined in RNA-seq experiments. (a) Summary of differentially expressed genes inrbm25-1. (b) Heat map of differentially expressed genes inrbm25-1. Samples (rows) and genes (column) are hierarchically clustered via Pearson correlation. (c) GO term distribution of differentially expressed genes inrbm25-1.(d) Validation of differential gene expression portion of the RNA-seq results by qRT–PCR analysis. Values represent mean±s.d. (n=3). Figure 4: The rbm25-1 mutation causes disrupted gene expression as determined in RNA-seq experiments. ( a ) Summary of differentially expressed genes in rbm25-1 . ( b ) Heat map of differentially expressed genes in rbm25-1 . Samples (rows) and genes (column) are hierarchically clustered via Pearson correlation. ( c ) GO term distribution of differentially expressed genes in rbm25-1. ( d ) Validation of differential gene expression portion of the RNA-seq results by qRT–PCR analysis. Values represent mean±s.d. ( n =3). Full size image RBM25 regulates the splicing of pre-mRNAs RBM25 has similar functional domains as the human splicing factor HsRBM25. To determine whether RBM25 functions in pre-mRNA splicing, we examined our RNA-seq data sets to look for potential effects of rbm25-1 mutation on pre-mRNA splicing. The analysis revealed that 359 genes have splicing defects in untreated rbm25-1 , while 416 genes show splicing defects in ABA-treated rbm25-1 ( Fig. 5a ; Supplementary Data 3 ). Our RNA-seq data analysis further revealed that the rbm25-1 mutation causes defects in splicing of gene transcripts in eight different alternative splicing categories: alternative acceptor, alternative donor, cassette exon, intron retention (IR), coordinate cassette exon, alternative first exon, alternative last exon and mutually exclusive exon ( Fig. 5b ; Supplementary Data 3 ). We designed primers unique to the intron of genes that are retained in the rbm25-1 plants and carried out semi-qRT–PCR assays to validate the IR results from the RNA-seq analysis. For RT–PCR analysis, we selected At4g16143 , At5g09330 , At2g42010 , At3g53340 , At4g32040 and At4g35800 . At4g16143 encodes importin alpha isoform 2. At5g09330 encodes NAC domain-containing protein 82. At4g42010 encodes phospholipase D beta 1. At3g53340 encodes nuclear factor Y, subunit B10. At4g32040 encodes KNOTTED1-like homeobox gene 5. At4g35800 encodes the unique largest subunit of nuclear DNA-dependent RNA II. The RT–PCR assays found that transcripts of At4g16143 , At5g09330 , At2g42010 , At3g53340 , At4g32040 and At4g35800 contain an intron in rbm25-1 and rbm25-2 with or without ABA treatment ( Fig. 5c,e ; Supplementary Fig. 3 ). Thus, the RT–PCR results confirmed the RNA-seq data of IR events in rbm25-1 . RT–PCR analysis confirmed that exon 4 of At2g48120 is skipped in rbm25 mutants under both control and ABA treatment conditions ( Fig. 5c ; Supplementary Figs 3 and 4 ). At2g48120 encodes the pale cress protein involved in chloroplast mRNA maturation [31] . 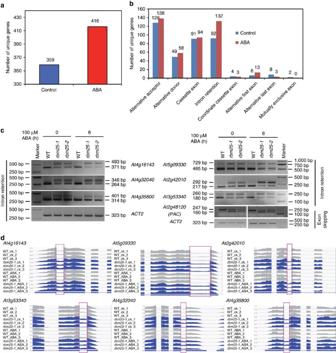Figure 5: Therbm25-1mutation causes defects in alternative splicing of gene transcripts. (a) Summary of genes whose transcripts were abnormally spliced inrbm25-1as determined by RNA-seq experiments. (b) Genes with defects in different types of alternative splicing patterns inrbm25-1as determined by RNA-seq experiments. (c) Validation of intron-retention and exon-skipping events in WT,rbm25-1andrbm25-2plants as determined by RT–PCR analysis. (d) Visualization with the integrative genomic viewer (IGV) of intron-retention events in WT andrbm25-1mutant plants. Annotated gene structures are shown (bottom), with thick lines representing exons and thin lines representing introns. Wiggle plots represent the normalized read coverage on an autoscale. Figure 5: The rbm25-1 mutation causes defects in alternative splicing of gene transcripts. ( a ) Summary of genes whose transcripts were abnormally spliced in rbm25-1 as determined by RNA-seq experiments. ( b ) Genes with defects in different types of alternative splicing patterns in rbm25-1 as determined by RNA-seq experiments. ( c ) Validation of intron-retention and exon-skipping events in WT, rbm25-1 and rbm25-2 plants as determined by RT–PCR analysis. ( d ) Visualization with the integrative genomic viewer (IGV) of intron-retention events in WT and rbm25-1 mutant plants. Annotated gene structures are shown (bottom), with thick lines representing exons and thin lines representing introns. Wiggle plots represent the normalized read coverage on an autoscale. Full size image The genes carrying defective alternative splicing patterns in rbm25-1 plants under control or ABA treatment conditions encode proteins with diverse functions in many biological processes, and the predicted roles of a good portion of these genes involve responses to abiotic or biotic stresses ( Supplementary Data 3 ). It is possible that altered activities of mis-spliced genes in unstressed rbm25-1 mutant account for differentially expressed genes in this mutant under control conditions as determined by RNA-seq analyses. There are 31 genes with a predicted role in DNA-dependent transcription in each category of abnormal splicing in unstressed rbm25-1 mutant ( Supplementary Data 3 ). These genes include promoter-specific transcription factors, general transcription factors and RNA polymerase II subunits. We reasoned that disrupted function of the mis-spliced genes in rbm25-1 plants should at least partly explain the impaired responses of rbm25 mutants to ABA treatment including alterations in gene expression and increased sensitivity of rbm25 mutants to ABA in terms of root growth and leaf yellowing. Thirty genes involved in transcription were found to have splicing defects in their transcripts in rbm25-1 mutant under ABA treatment ( Supplementary Data 3 ). These genes include the largest subunit of DNA-dependent RNA polymerase II, TATA-binding proteins, a nuclear factor, promoter-specific transcription factors and the subunits of the mediator complex. The mediators are involved in regulation of transcription from RNA polymerase II [32] . Loss-of-function or reduced activities of these genes will certainly lead to altered expression of genes in rbm25-1 mutant under ABA treatment. Although genes carrying splicing defects in rbm25-1 mutant under ABA treatment encode proteins involved in diverse biological processes, a substantial portion of the genes encode proteins that are predicted to function in biotic or abiotic stress-response pathways ( Supplementary Data 3 ). In addition, the calcium-sensing receptor and HAB1 are known regulators of ABA responses [33] , [34] , [35] . There are additional PP2Cs whose transcripts are mis-spliced in ABA-treated rbm25-1 mutant. Like HAB1, these PP2Cs may function as negative regulators of ABA signalling. Finally, impaired functions of four splicing factors (SC35-like splicing factor 33 encoded by At1g55310 , CC1-like splicing factor encoded by At2g16940 , U2 snRNP splicing factor encoded by At1g60900 and splicing endonuclease 1 encoded by At3g45590 ) may contribute to defects of alternative splicing of gene transcripts in rbm25-1 . ABA represses the expression of genes involved in photosynthesis including the small subunit of ribulose-1,5-bisphosphate carboxylase/oxygenase (Rubisco) ( rbcS genes) and chlorophyll a/b-binding proteins [36] , [37] . Related to this aspect of cellular function, we found mis-splicing of a group of genes that are involved in biogenesis and functionality of chloroplasts in ABA-treated rbm25-1 mutant. These genes include pale cress protein (encoded by At2g48120 ; the mutant of this gene has reduced chlorophyll content [31] ), the PsbQ subunit of the oxygen-evolving complex of photosystem II (encoded by At4g21280 ) [38] , starch branching enzyme 2.2 (encoded by At5g03650; it is transcriptionally regulated by the ABA-insensitive 4 (ABI4) [39] ), UDP-glycosyltransferase superfamily protein involved in flavonoid biosynthetic process (encoded by At4g09500 ) and plastid transcriptionally active 5 (PTAC5, encoded by At4g13670 (ref. 40 )) ( Supplementary Data 3 ). Mis-splicing for the transcripts of these proteins in rbm25-1 mutant may be associated or even contribute to the leaf yellowing phenotype of the mutant. Finally, we observed that a cyclin-dependent protein kinase (CDKC2 encoded by At5g64960 ) is mis-spliced in rbm25-1 under ABA treatment ( Supplementary Data 3 ). CDKC2 co-localizes with spliceosomal components in a manner dependent on the transcriptional status of the cells and on CDKC2-kinase activity. Expression of CDKC2 modifies the location of spliceosomal components [41] . Thus, disruption of CDKC2 may exacerbate the splicing defects caused by the rbm25-1 mutation. RBM25 controls the alternative splicing of HAB1 transcripts Our RNA-seq analysis revealed that the last intron of At1g72770 (which encodes HAB1) is retained in rbm25-1 plants ( Supplementary Data 3 ). HAB1 is one of the clade A PP2Cs that are co-receptors of ABA and important negative regulators of ABA signalling [14] , [33] , [42] , [43] . HAB1 transcripts are known to exist in three alternatively spliced forms (The Arabidopsis Information Resource, http://www.arabidopsis.org ). In our efforts to confirm intron-retention event in rbm25-1 and rbm25-2 with RT–PCR and qRT–PCR analyses, we found additional splicing defects of HAB1 in the rbm25 mutants. The rbm25 mutations cause altered accumulation of four alternatively spliced transcripts of HAB1 under control and ABA treatment conditions ( Fig. 6a,b ). Because HAB1 is upregulated by ABA, the defects of HAB1 are more pronounced in these two mutants under ABA treatment. In rbm25-1 and rbm25-2 plants, HAB1.1 ( At1g72770.1 ) displayed reduced expression level, while HAB1.2 ( At1g72770.2 ) and HAB1.4 ( At1g72770.4 , a previously unannotated splicing variant) showed increased expression level ( Fig. 6a,b ). The HAB1.2 and HAB1.4 isoforms are the intron-retained HAB1 transcripts identified in our RNA-seq experiments ( Supplementary Data 3 ). The expression level of HAB1.3 ( At1g72770.3 ) is very low and there is no difference between the wild type and rbm25 mutants for the accumulation of HAB1.3 transcripts ( Fig. 6b ). Transcripts of HAB1.2 and HAB1.4 will likely produce non-functional, truncated polypeptides of HAB1 ( Fig. 6c ). Therefore, the overall manifestation of the defect in HAB1 transcripts in rbm25-1 and rbm25-2 is the substantial reduction of HAB1.1 , the major transcript of HAB1 in wild-type plants ( Fig. 6b,c ). 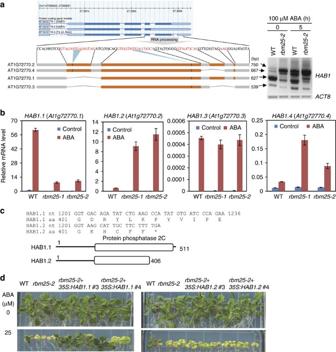Figure 6: RBM25 controls alternative splicing ofHAB1. (a) Different alternative splicing variants ofHAB1in WT andrbm25-2plants as determined by RT–PCR analysis followed by sequence analyses of cloned PCR products.ACT8was used as the loading control. In the close-up view of the portion corresponding to most parts of the last two exons ofAt1g72770.1, grey-shaded and orange-shaded boxes represent sequences in an exon, and folded lines between two boxes indicate introns in gene models ofAt1g72770.1,At1g72770.3andAt1g72770.4. (b) Relative transcript levels of different alternative splicing variants ofHAB1(expression level ofAt1g72770.1in unstressed WT was set to 1) in WT,rbm25-1andrbm25-2plants subjected to 100 μM ABA for 0 or 6 h as determined by qRT–PCR analysis. Values are mean±s.d. (n=4). (c) Deduced C-terminal portion of HAB1.1 and HAB1.2. The predicted domain structures of HAB1.1 and HAB1.2 (HAB1.4 has the same structure as HAB1.2) are also presented. (d) Effect ofHAB1on ABA sensitivity ofrbm25-1mutant plants. Five-day-old seedlings grown in MS medium were transferred to MS medium containing 0 or 25 μM ABA and grown for an additional 20-day period. Figure 6: RBM25 controls alternative splicing of HAB1 . ( a ) Different alternative splicing variants of HAB1 in WT and rbm25-2 plants as determined by RT–PCR analysis followed by sequence analyses of cloned PCR products. ACT8 was used as the loading control. In the close-up view of the portion corresponding to most parts of the last two exons of At1g72770.1 , grey-shaded and orange-shaded boxes represent sequences in an exon, and folded lines between two boxes indicate introns in gene models of At1g72770.1 , At1g72770.3 and At1g72770.4 . ( b ) Relative transcript levels of different alternative splicing variants of HAB1 (expression level of At1g72770.1 in unstressed WT was set to 1) in WT, rbm25-1 and rbm25-2 plants subjected to 100 μM ABA for 0 or 6 h as determined by qRT–PCR analysis. Values are mean±s.d. ( n =4). ( c ) Deduced C-terminal portion of HAB1.1 and HAB1.2. The predicted domain structures of HAB1.1 and HAB1.2 (HAB1.4 has the same structure as HAB1.2) are also presented. ( d ) Effect of HAB1 on ABA sensitivity of rbm25-1 mutant plants. Five-day-old seedlings grown in MS medium were transferred to MS medium containing 0 or 25 μM ABA and grown for an additional 20-day period. Full size image Ectopic expression of HAB1 suppresses rbm25-1 Loss-of-function mutations in HAB1 cause ABA hypersensitivity in early seedling growth and development [14] , [33] , [44] . Consistent with previous reports, the hab1-1 mutant is hypersensitive to ABA during seed germination and early seedling development ( Fig. 3b ). We observed that in response to ABA treatment hab1-1 mutant seedlings exhibit a leaf yellowing phenotype similar to that of rbm25 mutants, although the yellowing is not as severe as in rbm25 ( Fig. 2d ). Considering the central role of HAB1 in ABA signalling and the seedling growth and development phenotypes of hab1-1 mutant plants in response to ABA treatment, we hypothesized that the defects in HAB1 pre-mRNA splicing, particularly the dramatic reduction in HAB1.1 , may partially explain the leaf yellowing phenotype of ABA-treated rbm25 mutant plants. To test this hypothesis, we ectopically expressed full-length HAB1.1 complementary DNA (cDNA) under the CaMV 35S promoter in rbm25-2 mutant plants. As a control, we also expressed HAB1.2 cDNA under the CaMV 35S promoter in rbm25-2 mutant plants. Two independent lines of T 2 transgenic rbm25-2 seedlings were tested on media supplemented with 25 μM ABA. The results show that the ectopic expression of HAB1.1 but not HAB1.2 could partially rescue the leaf yellowing phenotype of rbm25-2 in response to ABA treatment ( Fig. 6d ). These results indicated that the HAB1.1 but not the HAB1.2 spliced form is functional in controlling leaf development under ABA treatment and the reduction of the HAB1.1 form contributes significantly to the leaf yellowing phenotype of rbm25 mutant plants. ABA affects splicing of transcripts We also examined the effect of ABA on the splicing pattern of transcripts in wild-type plants. ABA induces alternative splicing events in the transcripts of 27 genes in wild-type plants ( Supplementary Data 3 ). Among these alternatively spliced genes in ABA-treated wild-type plants, two of them ( At3g28670 and At3g24170 ) showed more severe splicing defects in ABA-treated rbm25-1 mutant. These results show that the ABA treatment causes defects in alternative splicing of pre-mRNAs in wild-type plants, and the splicing defects become much more severe when the splicing factor RBM25 is impaired. ABA regulates RBM25 transcript level and post-translationally ROA1 expression is upregulated by ABA treatment ( Fig. 7a ). This is consistent with publicly available gene expression profiling data on ROA1 under ABA treatment obtained using whole genome tiling arrays [45] ( Supplementary Fig. 5 ). This is also consistent with the ABA-induced mutant phenotypes and more severe splicing defects in rbm25 mutants under ABA treatment ( Supplementary Data 3 ), and suggests a need for more RBM25 to strengthen pre-mRNA splicing under ABA treatment. 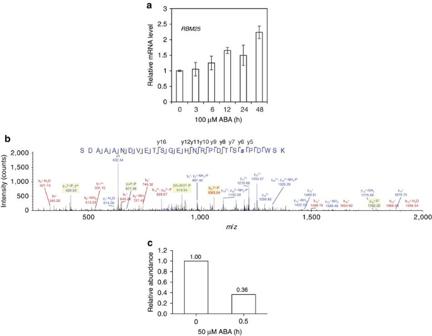Figure 7:RBM25is upregulated by ABA and ABA represses phosphorylation level of RBM25. (a) Relative transcript levels ofRBM25in WT plants as determined by qRT–PCR analysis. Values are mean±s.d. (n=4). (b,c) Quantitative phosphoproteomic profiles of total proteins were performed as described46. Proteins were extracted from 12-day-old WT plants subjected to 50 μM ABA treatment for 0 or 0.5 h, and the enrichment of the phosphoproteins and label-free quantification were performed as described46. This experiment was repeated three times with similar results. (b) Mass spectrometric spectra of a phosphopeptide (aa 407–432) in RBM25 identifiedin vivo. (c) Relative abundance of the RBM25 phosphopeptide. Figure 7: RBM25 is upregulated by ABA and ABA represses phosphorylation level of RBM25. ( a ) Relative transcript levels of RBM25 in WT plants as determined by qRT–PCR analysis. Values are mean±s.d. ( n =4). ( b , c ) Quantitative phosphoproteomic profiles of total proteins were performed as described [46] . Proteins were extracted from 12-day-old WT plants subjected to 50 μM ABA treatment for 0 or 0.5 h, and the enrichment of the phosphoproteins and label-free quantification were performed as described [46] . This experiment was repeated three times with similar results. ( b ) Mass spectrometric spectra of a phosphopeptide (aa 407–432) in RBM25 identified in vivo . ( c ) Relative abundance of the RBM25 phosphopeptide. Full size image Protein phosphorylation is central to ABA signalling [18] , [20] , [23] . ABA increases the phosphorylation levels of several splicing factors including arginine/serine-rich splicing factor 41, a PWI domain-containing protein, splicing factor U2af small subunit A and serine/arginine-rich protein splicing factor RSZ32, while ABA also represses the phosphorylation levels of several splicing factors [26] . Because RBM25 is upregulated by ABA, we examined whether phosphorylation status of RBM25 may also be regulated by ABA. We used a novel mass-spectrometry-based label-free quantitation method that facilitates systematic profiling of plant phosphoproteome changes with high efficiency and accuracy [46] . This method employs synthetic peptide libraries tailored specifically as internal standards for complex phosphopeptide samples and accordingly, a local normalization algorithm, LAXIC, which calculates phosphopeptide abundance normalized locally with co-eluting library peptides. Our mass-spectrometry studies revealed that RBM25 is phosphorylated and ABA represses the phosphorylation level of RBM25 ( Fig. 7b,c ). Based on this data, we suggest that dephosphorylation of RBM25 may be important for its splicing function under ABA treatment. Alternatively, dephosphorylation of RBM25 may be important for its protein stability because phosphorylation often leads to protein degradation through ubiquitin-mediated proteolysis [47] , [48] . In our unique genetic screen for regulators of ABA responses at seedling developmental stage, we identified a splicing factor, RBM25. The rbm25 mutant plants do not exhibit obvious growth and developmental defects under normal growth conditions, and the mutants are not altered in their responses to heat stress, ethylene or auxin. We established the identity of RBM25 through a map-based cloning strategy followed by a gene complementation analysis. Our genetic evidence demonstrated that RBM25 is required for proper ABA responses in plants by maintaining proper patterns of splicing of gene transcripts. Although splicing is important for all cellular processes involving gene expression, the splicing factor RBM25 is essential for root growth and leaf development in response to ABA but appears not to be required for normal growth and development. The rbm25 mutants are hypersensitive to ABA in the growth medium, indicating that RBM25 may be involved in mediating signal transduction events downstream of ABA. Indeed, our RNA-seq analyses revealed that RBM25 controls the splicing of one of the central ABA signalling molecules, HAB1 ( Fig. 6 ). Ectopic expression of HAB1.1 alone can partially suppress the hypersensitive phenotype of rbm25-2 to ABA in growth medium ( Fig. 6 ). These results indicate that RBM25 is critical for ABA signalling. Because gene splicing is an essential cellular process, it is difficult to obtain and study null alleles of splicing factor genes due to their lethality. The rbm25-1 and rbm25-2 alleles appear to be null alleles since RBM25 is not expressed in rbm25-1 and the PWI domain, which is presumably important for splicing function, is truncated in rbm25-2 ( Fig. 2b,f ). To our knowledge, this is the first time null alleles of a conserved splicing factor are found and characterized in plants. The conditional phenotype (that is, under ABA treatment only) of rbm25 mutants implies that RBM25 is not essential for splicing for all or most plant genes. However, there are some splicing defects in rbm25 mutant plants even under control conditions, but the splicing defects become more severe under ABA treatment such that growth and developmental phenotypes are manifested by the mutants under ABA treatment. Because rbm25 mutants lack obvious growth and developmental defects in the absence of ABA or in responses to heat stress and two additional hormones (ethylene and auxin), but have severe phenotypic defects in the presence of ABA ( Fig. 1 and Supplementary Fig. 1 ), we propose that plants may have a particular requirement for splicing in the presence of ABA. Indeed, this splicing factor (RBM25) shows increased expression under ABA treatment, which is consistent with the notion of an exaggerated requirement for splicing in the presence of ABA. On the other hand, we speculate that ABA signalling also regulates splicing in at least two ways: to increase the level of RBM25 transcript; and regulate the phosphorylation status of RBM25 ( Fig. 7 ; Supplementary Fig. 5 ) and other splicing factors [26] . The phosphorylation levels of several splicing factors are regulated by ABA in wild-type plants [26] , which perhaps strengthen splicing so as to help plant cope with ABA and related environmental stress. In this study, we showed that the phosphorylation level of RBM25 is downregulated by ABA and we propose that reduced phosphorylation of RBM25 might be important for its activity as a splicing factor or its protein stability under ABA treatment although the physiological significance of RBM25 phosphorylation remains to be determined. Because orthologues of RBM25 exist in various plant species ( Fig. 2c ; Supplementary Fig. 2 ), the molecular function of RBM25 may be conserved in other plant species including crops. Our RNA-seq experiments detected many genes whose splicing is controlled by RBM25. We observed that the rbm25-1 mutant plants carry splicing defects in alternative splicing of pre-mRNAs ( Supplementary Data 3 ). Our observation that there are more genes with defective splicing patterns when rbm25-1 mutant was treated with ABA is consistent with ABA upregulation of ROA1 ( Fig. 7a ; Supplementary Fig. 5 ; Supplementary Data 3 ). Intron-retained transcripts in rbm25-1 mutant tend to include premature stop codons and therefore produce truncated or even inactive forms of proteins. In addition, many IR events may lead to the generation of nonsense-mediated decay substrates so that the overall level of the transcript would decrease and no translation would take place. Other abnormal, alternatively spliced transcripts in rbm25-1 mutant probably produce non-functional proteins, and such splicing events were seldom detected in wild-type plants in our RNA-seq experiments. Several previous studies have shown that mutants with altered sensitivity to ABA are affected in pre-mRNA splicing under normal developmental conditions [49] , [50] , [51] , [52] , [53] , [54] , [55] or under abiotic stress conditions including drought and salinity [56] , [57] , [58] , [59] , [60] . In the previous studies, the various mutants were defective in ABA-regulated seed germination and/or stomatal regulation, but not in seedling leaf greening. In addition, the previously published mutants are defective in not only splicing but also other RNA processing events, and the published work did not link the mis-splicing of a particular gene(s) to the mutant phenotypes. In contrast, the rbm25 mutants are primarily defective in leaf greening in response to ABA, and we have identified the mis-splicing of HAB1 as a critical mis-spliced gene contributing to the mutant phenotype ( Fig. 6 ), although the defective splicing in many other genes may also contribute to the mutant phenotypes of rbm25 . Plant materials T-DNA insertional mutant pool with known T-DNA insertion sites including rbm25-1 (SALK_064472) were obtained from Arabidopsis Biological Resource Center (ABRC; Columbus, OH). rbm25-2 (containing pTCH4:LUC reporter gene [29] ; seeds of pTCH4:LUC line was kindly provided by Dr Janet Braam) was isolated from a T-DNA-mutagenized Arabidopsis T 2 population. Seeds were surface sterilized and sown in germination medium (1 × Murashige–Skoog (MS) salts, 2% sucrose, 1.2% agar, pH 5.7). For ABA-sensitivity screening, 5-day-old seedlings were transferred to new MS agar plates supplemented with 5 μM ABA and were allowed to grow vertically for an additional 15–20 days. Seeds of hab1-1 (SALK_002104) were obtained from the ABRC. Plants at all developmental stages were grown in a growth chamber at 22±1 °C under cool, white light ( ∼ 100–120 μmol m −2 s −1 ) with a long-day photoperiod (16-h light/8-h dark). Map-based cloning and gene complementation The rbm25-1 mutant was crossed with the Landsberg erecta accession, and a total of 896 plants homozygous for the rbm25-1 phenotype in response to ABA in MS medium were selected from the F 2 population. A separate F 2 population was also generated from a cross between rbm25-2 and Landsberg erecta , and 896 plants homozygous for the rbm25-2 phenotype in response to ABA in MS medium were selected. Simple sequence length polymorphism markers were designed according to the information in the Cereon Arabidopsis Polymorphism Collection and were used to analyse recombination events. Mapping indicated that rbm25-1 and rbm25-2 mutations were located on the BAC clones T30E16 and F8A5. Candidate genes within this region were sequenced from the rbm25 mutants and compared with those in GenBank to find the rbm25-1 and rbm25-2 mutations. For gene complementation of roa1 mutants, a 7.4-Kb genomic fragment of At1g60200 including 2.2 Kb upstream of the translation initiation codon and 0.4 Kb downstream of the translation initiation codon was amplified by PCR with T13D8 as a template (primers were listed in Supplementary Data 1 ). The amplified fragment was first cloned via Gateway technology (Invitrogen) into the pENTR1A Dual Selection Vector. The RBM25 gene was then introduced into the pGWB501 vector, resulting in plasmid pGWB501-ROA1. The pGWB501-ROA1 construct was transferred into Agrobacterium tumefaciens (strain GV3101), and rbm25-1 and rbm25-2 plants were transformed by the floral dip method. Transgenic plants were selected on MS agar plates containing 50 mg l −1 hygromycin. Subcellular localization The ∼ 2-Kb genomic DNA fragment upstream of the start codon of RBM25 ( At1g60200 ) was amplified by PCR with T13D8 as a template using the primer pair At1g60200P-F5 and At1g60200P-R2, resulting in DNA fragment I. The coding region of At1g60200 (from the start codon to the last codon without stop codon or any intron sequences) was amplified by PCR with the primer pairs At1g60200CDS-F2 and At1g60200CDS-R2, resulting in DNA fragment II. The DNA fragments I and II were joined together by PCR amplification using the primer pairs At1g60200P-F5 and At1g60200CDS-R2 with DNA fragments of I and II as a template. The resulting DNA fragment III was cloned into a vector pENTR1A initially and subsequently into the binary vector pGWB504, resulting in the plasmid RBM25:RBM25–GFP. The RBM25:RBM25–GFP construct was then introduced into Arabidopsis wild-type (Col-0) plants by floral dip transformation with A. tumefaciens strain GV3101. The subcellular localization of RBM25:RBM25–GFP protein in roots of transgenic plants (T 2 generation) was determined with a Leica SP5X confocal microscope (Leica Microsystems). Construction of the 35S:HAB1.1 and 35S:HAB1.2 plasmids The cDNA fragments were amplified by PCR with primer pairs HAB1CD-F1 plus HAB1CD-R1 (for HAB1.1 ) and HAB1CD-F1 plus HAB1CD-R2 (for HAB1.2 ). The amplified cDNA fragments were initially cloned into the vector pENTR-D/TOPO and subsequently into the binary vector pGWB2 to generate plasmids 35S:HAB1.1 and 35S:HAB1.2. These plasmids were then introduced into Arabidopsis wild-type (Col-0) plants into rbm25-2 plants by floral dip transformation with A. tumefaciens strain GV3101. RNA-seq data analyses and validation experiments Fourteen-day-old wild-type and rbm25-1 seedlings grown on MS medium (1 × MS salts, 2% sucrose, 0.6% agar, pH 5.7) were treated with 0 or 100 μM ABA for 6 h and were used for total RNA extraction. Total RNA was isolated with the Universal Plant Total RNA Extraction Kit (BioTeke) and treated with TURBO DNA-free Kit (Ambion) to remove any genomic DNA contaminants. mRNA-seq libraries were constructed following the standard Illumina protocols. There are three biological replicates per genotype. Illumina sequencing was performed in the Shanghai Center for Plant Stress Biology with an Illumina HiSeq 2500 System. For each sample, RNA-seq raw reads were trimmed using Trimmomatic v0.32 and PRINSEQ v0.20.4 (refs 61 , 62 ). Trimmomatic was used to remove the potential Illumina adapter contamination and conduct read trimming and clipping the low quality bases. PRINSEQ was subsequently employed to mainly remove low-complexity reads. The remained reads were then aligned to A. thaliana genome sequence and the reference-annotated genes (TAIR10) using TopHat v2.0.13 programme [63] with customized parameters specially for our RNA-seq libraries from plant A. thaliana (--read-edit-dist 3--read-realign-edit-dist 0--b2-very-sensitive-r 150--mate-std-dev 200-a 6-i 8-I 10000--min-segment-intron 8--max-segment-intron 10000--microexon-search). According to RNA-seq-mapped reads and the reference-annotated transcripts, transcriptomes were reconstructed for each sample by Cufflinks v2.2.1 (ref. 64 ). Given variable efficiency of mRNA enrichments and rRNA depletion kits in samples, these transcripts were masked in transcriptome constructions to improve the overall robustness of transcript abundance estimates. To obtain a high confidence of transcriptomes, the novel constructed transcript was filtered out when the abundance was <20% (default is 10%) of the most abundant isoform for each gene. Then all of the constructed transcriptomes were merged with the reference-annotated transcripts using Cuffmerge [64] to yield comprehensive re-annotated gene transcripts including known and novel annotated transcripts in our RNA-seq samples. Subsequently, significantly differentially expressed genes were predicted by Cuffdiff [64] between the controls and tested samples, using twofold change and multiple test P value<0.05. Given that IR is the most frequent alternative splicing (AS) type in plants [65] , [66] and juncBASE especially improves the reliability of the detection for such AS type [67] , we adopted juncBASE v0.6 to identify AS events within genes for our samples. First, two different databases were constructed, one is based on comprehensive re-annotated gene transcripts (as described above) to identify all internal AS events (not alternative first or last exon events), and the other is derived from just the reference-annotated transcripts to define alternative first and last exons. Then, a series of python scripts from juncBASE were employed to identify exon–exon junctions, exon–intron junctions and AS events, qualify the events and give significantly differentially splicing events between samples. Accordingly, juncBASE-detected AS events ranged from ∼ 15,500 to ∼ 20,500, and among the events 358 to 1,464 ones showed significantly differentially AS events ( P value<0.05 and abs (delta_val)>5) between pair-wise samples. Moreover, a module from CASH (comprehensive alternative splicing hunting, the renewed version of ASD (alternative splicing detector [68] ) was used to rescue 19 to 50 differential IR events. Only genes with alternative splicing patterns in all three biological replicates of rbm25-1 mutant plants are listed as differentially alternatively spliced genes. For RT–PCR and qRT–PCR analyses, 5 μg of total RNA was used for synthesis of the first-strand cDNA. Each experiment had three to four biological replicates and was repeated at least three times. The comparative cycle threshold (ct) method was applied for calculating gene expression levels, and ACT2 was used as a reference gene. Accession codes: The RNA-seq data have been deposited in NCBI Gene Expression Omnibus (GEO) database under the accession code GSE66737 . How to cite this article: Zhan, X. et al . An Arabidopsis PWI- and RRM motif-containing protein is critical for pre-mRNA splicing and ABA responses. Nat. Commun. 6:8139 doi: 10.1038/ncomms9139 (2015).